Mesopore quality determines the lifetime of hierarchically structured zeolite catalysts Deactivation due to coking limits the lifetime of zeolite catalysts in the production of chemicals and fuels. Superior performance can be achieved through hierarchically structuring the zeolite porosity, yet no relation has been established between the mesopore architecture and the catalyst lifetime. Here we introduce a top-down demetallation strategy to locate mesopores in different regions of MFI-type crystals with identical bulk porous and acidic properties. In contrast, well-established bottom-up strategies as carbon templating and seed silanization fail to yield materials with matching characteristics. Advanced characterization tools capable of accurately discriminating the mesopore size, distribution and connectivity are applied to corroborate the concept of mesopore quality. Positron annihilation lifetime spectroscopy proves powerful to quantify the global connectivity of the intracrystalline pore network, which, as demonstrated in the conversions of methanol or of propanal to hydrocarbons, is closely linked to the lifetime of zeolite catalysts. The findings emphasize the need to aptly tailor hierarchical materials for maximal catalytic advantage. The industrial viability of heterogeneously catalysed processes is often severely constrained by catalyst deactivation. In practice, alongside sintering and poisoning, fouling due to coke deposition is one of the principal causes of deactivation [1] . Besides an appropriate choice of reactor configuration and process conditions, an effective means to retard losses of activity and/or selectivity due to coking is by tuning the catalyst properties [2] , [3] . In this context, there are still great incentives to improve the intrinsic stability of zeolite catalysts, owing to their widespread application as solid acids in, for example, fluid catalytic cracking, methanol upgrading, the oligomerization or aromatization of light olefins, alkylation reactions and so on [3] . Numerous recent studies have demonstrated substantial prolongations of the lifetime of zeolite catalysts upon provision of a secondary network of meso- and/or macropores. This can be achieved by decreasing the crystal size in one or more dimensions (termed nanosized zeolites) [4] , [5] , [6] or by creating intracrystalline mesopores through templating or demetallation strategies (termed hierarchical zeolites) [7] , [8] . An improved resistance to coking with increasing external (mesopore) surface area can be envisaged due to the facilitated escape of coke precursors and the larger area that needs to be covered to block access to the micropores [9] , [10] , [11] , [12] . A question of urgent relevance is how the quality of the mesopores, determined by their size, distribution, and connectivity in the crystals impact their ability to enhance the catalytic performance. One of the foremost challenges in addressing this most overlooked aspect is the identification of samples with comparable absolute porosity and acidity, but distinct mesopore topology. Furthermore, advanced space- and time-resolved characterization tools are essential to access, localize and quantify nanostructural details of the hierarchical arrangement [13] , [14] . Base leaching offers a simple, versatile and scalable means to prepare hierarchical zeolites with well-defined properties [15] . Porosity modification can be tuned through the inclusion of additives, such as quaternary ammonium or metal salts, to the alkaline solution. Since the size and amount of developed mesopores can be regulated by the identity and concentration of additive applied, they are commonly referred to as pore-directing agents [16] . In the case of ZSM-5 zeolites, tetrapropylammonium cations (TPA + ) are known to provide a high level of control over the dissolution process due to their strong interaction with the crystal surface [17] . On the basis of our growing experience with the application of this pore-directing agent, we hypothesize that the action of TPA + could be exploited to synthesize and consequently verify the performance of hierarchical ZSM-5 zeolites with distinct intracrystalline mesopore topology. Furthermore, since the quality of the mesopore network can vary widely depending on the synthesis approach, the resulting demetallated samples are contrasted with hierarchical zeolite structures attained via the well-known bottom-up strategies of carbon templating [18] , [19] and seed silanization [20] , [21] . To corroborate this, we draw on porosity techniques and seek advanced microscopic and spectroscopic methods to fully discriminate the pore structures and acidic properties. In particular, we demonstrate the powerful combination of correlative scanning transmission-secondary electron imaging coupled with positron annihilation lifetime spectroscopy for the comprehensive characterization of materials with complex multipore networks. The instrumental impact of the mesopore architecture on the lifetime of the zeolites is evaluated in the upgrading of methanol or of propanal to hydrocarbons, notorious coke-forming reactions of great practical significance [12] , [22] , [23] , [24] . Hierarchical structuring of ZSM-5 zeolites To assess the impact of mesopore architecture on the catalyst lifetime in coke-forming reactions, it was first necessary to identify hierarchical zeolites with comparable bulk characteristics among the samples attained by the bottom-up (demetallation) and top-down (carbon templating and seed silanization) methods. The preparation of hierarchical zeolites by demetallation involved the post-synthetic treatment of a purely microporous zeolites (coded C) in aqueous sodium hydroxide (resulting in H1 zeolites) or by analogous treatment in the presence of tetrapropylammonium bromide (yielding H2 zeolites). In this instance, we expected that by applying elevated concentrations of TPA + we could purposefully drive the preferential dissolution of internal parts of the crystal while achieving a similar extent of mesoporosity. Two commercial ZSM-5 zeolites with respective nominal bulk Si/Al ratios of 40 (Z40-C) and 50 (Z50-C) were studied to verify the impact of compositional and morphological differences on the homogeneity of mesopore development at the crystal level. Hierarchical zeolites prepared by the bottom-up approaches of carbon templating (coded CT1) and seed silanization (coded SS) were synthesized by established protocols. In the former method, the crystallization of the zeolite in the presence of a carbon matrix results in the formation of meso-/macropores upon subsequent removal of the template by combustion [18] , [19] . In contrast, the latter method relies on the self-assembly of seed-silanized nanounits formed by the inclusion of organosilane molecules (in this case phenylaminopropyltrimethoxysilane, PHAPTMS) into the synthesis gel. The organosilanes serve a dual purpose, both perturbing the growth of the zeolite crystals and increasing the porosity of the resulting hierarchical zeolite on their removal [20] , [21] . An additional carbon-templated zeolite, kindly provided by Haldor Topsøe (coded CT2), was evaluated for comparative purposes. Examination of the high-resolution transmission electron microscopy (TEM) images highlights the distinctive structures of the resulting ZSM-5 catalysts ( Fig. 1 ). As expected, the development of intracrystalline mesopores is evident on alkaline treatment of the conventional Z50-C. Herein, the starkly different appearance of Z50-H1 and Z50-H2 is of unique interest; in contrast, with the heavily leached surface displayed by the former, well-preserved crystal facets and discrete homogeneously distributed mesopores in the latter are consistent with the expected pore-directing impact of the tetrapropylammonium cations. In contrast, the crystal morphology of the hierarchical zeolites prepared by carbon templating and seed silanization routes is less defined. While intracrystalline mesopores of differing size are distinguished in the former samples, the latter zeolite displays predominantly intercrystalline mesopores, with small mesopores (3–4 nm) formed on the removal of the organosilane component coexisting with larger voids resulting from the self-assembly process. Analysis by X-ray diffraction confirms the presence of a single crystalline MFI phase in each case ( Supplementary Fig. 1 ). 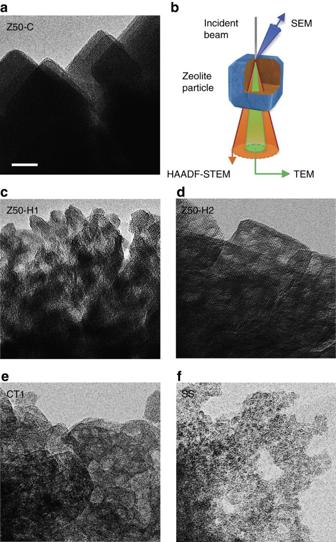Figure 1: Transmission electron microscopic examination of the zeolites. In comparison with the uniform contrast of the purely microporous crystals of a conventional ZSM-5 (Z50-C,a), the mesoporous nature of the hierarchical zeolites is clearly visible by TEM. Whereas intracrystalline mesopores are evidenced in the catalysts prepared by post-synthetic alkaline treatment (Z50-H1,cand Z50-H2,d) or by carbon templating (CT1,e), the synthesis by seed silanization (SS,f) resulted in the agglomeration of nanocrystals (around 5–10 nm in diameter) and extensive intercrystalline mesoporosity. Remarkably, the gaping fissures and jagged crystal edges exhibited by Z50-H1 zeolite relative to the more internally distributed discrete mesopores and the better preserved external surface of the crystals of Z50-H2 zeolite illustrate the directing role of TPA+in the preparation of the latter sample. The sketch inbshows the electron microscopic approach enabling the acquisition of information specific to the bulk (TEM, HAADF-STEM) or external surface (SEM) structure of a crystal. Scale bar indicates 20 nm and applies to all micrographs. Figure 1: Transmission electron microscopic examination of the zeolites. In comparison with the uniform contrast of the purely microporous crystals of a conventional ZSM-5 (Z50-C, a ), the mesoporous nature of the hierarchical zeolites is clearly visible by TEM. Whereas intracrystalline mesopores are evidenced in the catalysts prepared by post-synthetic alkaline treatment (Z50-H1, c and Z50-H2, d ) or by carbon templating (CT1, e ), the synthesis by seed silanization (SS, f ) resulted in the agglomeration of nanocrystals (around 5–10 nm in diameter) and extensive intercrystalline mesoporosity. Remarkably, the gaping fissures and jagged crystal edges exhibited by Z50-H1 zeolite relative to the more internally distributed discrete mesopores and the better preserved external surface of the crystals of Z50-H2 zeolite illustrate the directing role of TPA + in the preparation of the latter sample. The sketch in b shows the electron microscopic approach enabling the acquisition of information specific to the bulk (TEM, HAADF-STEM) or external surface (SEM) structure of a crystal. Scale bar indicates 20 nm and applies to all micrographs. Full size image Inspection of the compositional, porous and acidic properties quantitatively illustrates the diverse attributes of the hierarchically structured zeolites ( Table 1 ). Evaluation by nitrogen sorption coupled with appropriate models importantly verifies the similar bulk porous properties of the H1 and H2 zeolites. Interestingly, despite the distinct structure observed by TEM, the sample prepared by seed silanization displays a comparable mesopore surface area and volume to those of the demetallated zeolites, but a smaller mesopore diameter and a slightly increased micropore volume. In contrast, the carbon-templated zeolites exhibit a lower mesopore surface area (88 and 154 m 2 g −1 for CT1 and CT2, respectively) coinciding with those previously reported for hierarchical zeolites prepared via this method [25] . This relates well with the larger average mesopore diameter (>20 nm) of these materials in comparison with the alkaline-treated (5–10 nm) or seed-silanized ( < 5 nm) samples. Nonetheless, the hierarchical zeolites synthesized via carbon templating possess a mesopore volume almost three times that of the conventional ZSM-5. Table 1 Characterisation data of the zeolites. Full size table Assessment by the infrared study of adsorbed pyridine confirmed the remarkably comparable acidic properties of the H1 and H2 hierarchical zeolites derived from a particular conventional zeolite ( Table 1 ). As expected, a largely preserved number of Brønsted acid sites and an approximately four times increased concentration of Lewis acid sites are observed with respect to the purely microporous counterparts. However, the concentrations of Brønsted acid sites in the samples prepared by direct synthesis were noticeably lower than those of the demetallated analogues of similar bulk composition [26] . The differing Brønsted acid site density of the carbon-templated samples emphasizes the difficulty in obtaining two equivalent hierarchical zeolites even when following a similar approach. Consequently, in view of the closest correspondence in both porous and acidic properties, the H1 and H2 zeolite were identified as optimal samples to determine the impact of mesopore topology, and the characteristics of the pore network were characterized in depth. Porous and acidic attributes of the demetallated zeolites In relation to the type I isotherms evidenced for the conventional materials, the alkaline-treated zeolites exhibited combined type I–IV behaviour characteristic of the creation of extensive mesoporosity on desilication ( Fig. 2a and Supplementary Fig. 1 ). Compared with the parallel adsorption and desorption branches typical of open and channel-like mesopores observed for the standard alkaline-treated samples, the hierarchical zeolites prepared with TPA + displayed a prominent hysteresis with a closure point at p / p 0 =0.42. This suggests that a certain fraction of mesopores can only be assessed either through micropores (which we consider as occluded mesopores) or through entrances <4 nm in diameter (which we refer to as constricted mesopores) in the H2 samples [27] , [28] . In addition, a smaller average mesopore diameter of around 5 nm with respect to 8 nm resulted on inclusion of the pore-directing agent ( Table 1 ). 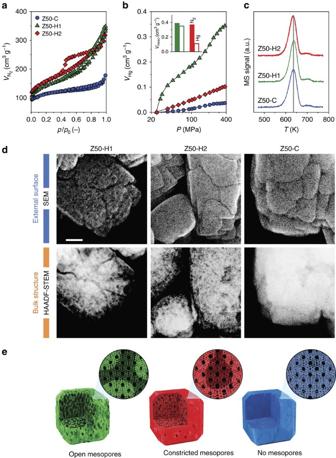Figure 2: Assessment of mesopore location in alkaline-treated zeolites. (a,b) A pronounced hysteresis in the nitrogen isotherm (a) and a significantly lower uptake in mesopores between 4 and 50 nm in size in the mercury intrusion curve (b) suggest a more internal nature of the mesopores in the hierarchical zeolite prepared in the presence of TPA+(Z50-H2) than that attained by the additive-free treatment (Z50-H1). Thus, only 30% of the mesopores detected by nitrogen were accessible to mercury in Z50-H2 in contrast to 90% for Z50-H1 (inset). (c) The equivalent temperature of the peak maximum in the evolution of propene observed during the TPSR ofn-propylamine, confirms the identical strength of Brønsted acid sites in the conventional and treated zeolites. (d) The distinct mesopore distribution within the hierarchical zeolites is unequivocally discriminated by identical-location SEM and HAADF-STEM imaging: the relatively preserved crystal surface of Z50-H2 observed in SE micrographs distinctly contrasts with the highly pitted surface of Z50-H1, appearing unaltered from that of the conventional zeolite; while the prominent regions of dark contrast observed in HAADF-STEM projections evidence the presence of extensive mesoporosity in both Z50-H1 and Z50-H2 compared with the solid appearance of Z50-C. (e) The distinct 3D structure of the open and constricted mesopores is illustrated schematically to facilitate visualization. Scale bar indicates 50 nm and applies to all micrographs. Figure 2: Assessment of mesopore location in alkaline-treated zeolites. ( a , b ) A pronounced hysteresis in the nitrogen isotherm ( a ) and a significantly lower uptake in mesopores between 4 and 50 nm in size in the mercury intrusion curve ( b ) suggest a more internal nature of the mesopores in the hierarchical zeolite prepared in the presence of TPA + (Z50-H2) than that attained by the additive-free treatment (Z50-H1). Thus, only 30% of the mesopores detected by nitrogen were accessible to mercury in Z50-H2 in contrast to 90% for Z50-H1 (inset). ( c ) The equivalent temperature of the peak maximum in the evolution of propene observed during the TPSR of n -propylamine, confirms the identical strength of Brønsted acid sites in the conventional and treated zeolites. ( d ) The distinct mesopore distribution within the hierarchical zeolites is unequivocally discriminated by identical-location SEM and HAADF-STEM imaging: the relatively preserved crystal surface of Z50-H2 observed in SE micrographs distinctly contrasts with the highly pitted surface of Z50-H1, appearing unaltered from that of the conventional zeolite; while the prominent regions of dark contrast observed in HAADF-STEM projections evidence the presence of extensive mesoporosity in both Z50-H1 and Z50-H2 compared with the solid appearance of Z50-C. ( e ) The distinct 3D structure of the open and constricted mesopores is illustrated schematically to facilitate visualization. Scale bar indicates 50 nm and applies to all micrographs. Full size image Alongside N 2 sorption, which probes the entire intracrystalline pore network, mercury porosimetry offers a unique advantage; since at the highest pressure (around 418 MPa) it can only penetrate mesopores down to around 4 nm in diameter, it can be applied to discriminate their relative accessibility from the crystal surface [29] , [30] . Herein, in spite of the identical mesopore volumes evidenced by N 2 sorption, the maximum intrusion of mercury was substantially reduced in zeolites prepared by the TPA + -modified treatment compared with that observed for zeolites obtained by the additive-free route ( Fig. 2b ). In fact, direct comparison reveals that while almost 90% of the mesopore volume determined by N 2 sorption is also accessible to mercury in Z50-H1, the fraction of accessible mesopores in Z50-H2 is only 30% ( Fig. 2b , inset). Consistent with the indications of nitrogen sorption, these findings directly suggest that the majority of mesopores in the hierarchical zeolites desilicated in the presence of TPA + are connected to the crystal surface via pores smaller than 4 nm. The predominance of constricted rather than occluded mesopores in Z50-H2 was substantiated by assessment through pore-plugging methods exploiting n -nonane [31] , [32] ( Supplementary Fig. 2 ). Complementing the equivalent concentrations of acid sites determined by the infrared study of adsorbed pyridine, the identical strength of Brønsted sites in the demetallated zeolites was verified by temperature-programmed surface reaction (TPSR) of n -propylamine ( Fig. 2c ). We previously demonstrated the sensitivity of this technique to the variation in the acid strength of post-synthetically modified ZSM-5 zeolites [33] . The amount of propene formed on the decomposition of n -propylamine adsorbed in stoichiometric quantities on Brønsted acid sites is consistent with the similar amount of acid sites determined by the pyridine adsorption in the alkaline-treated zeolites ( Supplementary Fig. 3 ). Visualization of the mesopore distribution To gain improved insight into the accessibility of the mesopores in the demetallated zeolites, our efforts turned to visualizing the samples by electron microscopy in different imaging modes ( Fig. 1b ). While the high-resolution TEM images had indicated a higher fraction of mesopores connected with the external surface in Z50-H1 compared with Z50-H2 ( Fig. 1c,d ), spatial information is inevitably lost when the structural features of a 3D object are overlaid in a 2D image unless methods are used to retrieve this in the third dimension, such as through the application of TEM tomography [34] , [35] , [36] . However, the versatility of this extremely powerful technique is somewhat limited by the substantial time required for data acquisition and post-processing. We have taken another route by using an aberration-corrected scanning transmission electron microscope (STEM) to record identical-location secondary electron (SE) and high-angle annular dark-field (HAADF) signals [37] , [38] , [39] . An SE detector installed within the condenser of an STEM microscope permits high-resolution examination of the morphology of individual zeolite particles, thereby providing correlative insight into the impacts of demetallation on both the external and bulk structure. Although exceptional works have demonstrated the value of this technique for the spatial localization of supported metal nanoparticles [37] , [38] and to confirm the pore uniformity in ordered mesoporous silicas [39] , its applicability to assess the distribution of porosity levels in complex hierarchical materials has not been previously investigated. Decisively, the prominent observation of large open mesopores in the SE micrographs of the heavily eroded external crystal surface of the H1 zeolite contrast with the few readily distinguishable mesopores and pristine appearance of the crystal surface of the H2 sample, which appeared identical to that of the conventional zeolite ( Fig. 2d and Supplementary Fig. 4 ). The creation of extensive intracrystalline mesoporosity in both the H1 and H2 zeolites could be readily distinguished from the areas of dark contrast in the HAADF-STEM images, in comparison with the uniform bright contrast observed for the conventional zeolite. These findings corroborate the respective introduction of open and constricted mesopores in the hierarchical H1 and H2 zeolites (illustrated schematically in Fig. 2e ), in agreement with the relative fraction of accessible mesopores probable by mercury in these samples. Quantification of mesopore network connectivity The catalytic performance of hierarchical zeolites is firmly expected to depend on the connectivity of the pore network and consequently on the mesopore architecture. However, despite the development of various methods based on microscopy, physisorption, spectroscopy and so on, determination of the pore network connectivity remains very difficult, particularly due to the distinct sensitivity of these techniques to the coexistence of micro- and mesopores [40] . To this end we explored the application of beam-based positron annihilation lifetime spectroscopy (PALS), a rapidly maturing non-destructive technique capable of probing the entire void volume [41] . PALS owes its sensitivity to the fact that ortho-positronium ( o -Ps) species formed in a solid on positron implantation are long-lived enough to diffuse through porous media, but rapidly lose energy on successive collisions with the pore surface and may be trapped decaying with a lifetime proportional to the pore size ( Fig. 3a ) [42] , [43] . Owing to its limited previous application for the characterization of hierarchically structured materials, a full description of the methodological approach explaining the experimental set-up, data acquisition and spectral analysis is provided in the supplementary information to improve the accessibility of this technique. 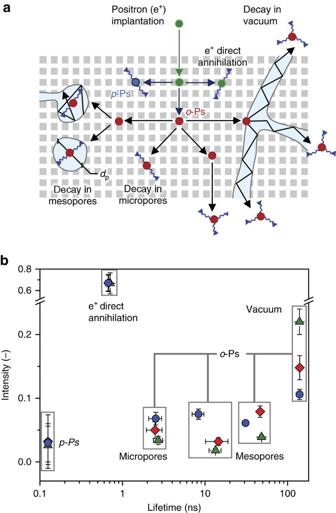Figure 3: Positron annihilation lifetime spectroscopy. (a) When positrons are implanted into a sample, they can directly annihilate into two gamma rays or may bind with electrons forming positronium; para-positronium (p-Ps) decays rapidly while the longer-lived ortho-positronium (o-Ps) can diffuse through porous solids and escape into vacuum or can decay with a lifetime proportional to the pore size (dp) due to the interaction with an electron other than that to which it is bound (the so called pick-off effect). (b) Spectral fitting reveals lifetime components representative of the ZSM-5 micropores (0.55 nm) and of mesopores between 3.3 and 12 nm for the conventional (Z50-C, circles) and hierarchical zeolites (Z50-H1, triangles and Z50-H2, diamonds). The fraction ofo-Ps escaping into vacuum relates to the interconnectivity of the micro- and mesopore network with the crystal surface (Z50-H1>Z50-H2>Z50-C). A χ2-statistical test was used and error bars indicate the s.d. Figure 3: Positron annihilation lifetime spectroscopy. ( a ) When positrons are implanted into a sample, they can directly annihilate into two gamma rays or may bind with electrons forming positronium; para-positronium ( p -Ps) decays rapidly while the longer-lived ortho-positronium ( o -Ps) can diffuse through porous solids and escape into vacuum or can decay with a lifetime proportional to the pore size ( d p ) due to the interaction with an electron other than that to which it is bound (the so called pick-off effect). ( b ) Spectral fitting reveals lifetime components representative of the ZSM-5 micropores (0.55 nm) and of mesopores between 3.3 and 12 nm for the conventional (Z50-C, circles) and hierarchical zeolites (Z50-H1, triangles and Z50-H2, diamonds). The fraction of o -Ps escaping into vacuum relates to the interconnectivity of the micro- and mesopore network with the crystal surface (Z50-H1>Z50-H2>Z50-C). A χ 2 -statistical test was used and error bars indicate the s.d. Full size image Six lifetime components were evidenced in the positron annihilation lifetime spectra of the conventional and hierarchical zeolites, which describe the final state of the system after diffusion and trapping ( Fig. 3b and Supplementary Table 1 ). The two shortest lifetimes, corresponding to the rapid decay of para-positronium ( p -Ps, 0.125 ns) and of free positrons (e + , 0.7 ns), are unrelated to the pore structure. In contrast, the contribution arising at around 2.6 ns is in excellent agreement with the lifetime expected for o -Ps in the micropores of the MFI framework [44] and that observed between 20 and 40 ns is in line with the presence of mesopores of ~\n3.3 nm (Z50-C), 8–12 nm (Z50-H1) and 4–6 nm (Z50-H2) in diameter (depending on the pore geometry assumed [45] ). While the estimated mesopore diameters of the hierarchical zeolites correlate well with those derived by gas sorption, the presence of mesopores in the conventional zeolite suggests the likely existence of isolated defects within the crystal aggregates. The fraction of o -Ps annihilating in the micro- and mesopores (Ps micro and Ps meso in Table 2 ) depends on both the respective pore volume and connectivity. The relatively high fraction of Ps micro observed for the conventional zeolites coincides with the longer diffusion path within the micropores. The physical origin of the component identified between 8 and 12 ns, which is suggestive of pores of 1.2–1.4 nm in diameter, is not yet clear. Interestingly, its fraction decreases following base leaching inferring the disappearance of structural defects contributing to this signal. Table 2 Positron annihilation lifetime spectroscopy data. Full size table The longest lifetime component corresponds to the self-annihilation of o -Ps in vacuum, and the contribution of this component (Ps vacuum ) relates to the probability of their escape from the intracrystalline pore network, with H1>H2>C ( Fig. 3b and Table 2 ). Since the movement of o -Ps from a micropore to a mesopore dominates over the reverse process, Ps vacuum strongly relates to the interconnection of the mesopores, and thus the observed trend coincides with our expectations. Interestingly, Z40-H2 displays higher values of Ps vacuum compared with that evidenced for the Z50-H2, which is tentatively ascribed to the greater surface roughness visible by SEM/HAADF-STEM ( Supplementary Fig. 5 ). The unprecedented sensitivity of PALS to gauge the bulk connectivity of the complex pore network in addition to discriminating the size of the pores, surpasses all other state-of-the-art techniques. In contrast to the demetallated zeolites, the efficiency of the mesopores to enhance o -Ps escape into vacuum was relatively low in the samples prepared by carbon templating and seed silanization ( Table 2 ). In the former case, the high fraction of o -Ps decaying in the zeolite micropores, which is similar to that in the conventional ZSM-5, is consistent with the decreased probability of o -Ps migration from micro- to mesopores owing to the moderate external surface area achieved in the presence of large mesopores. In the case of the latter, the high fractions of o -Ps annihilating in the micro- and mesopores suggest an increased resistance to migration both from micro- to mesopores and from the micro-/mesopores to vacuum. This would be expected if the diffusion length in a particular pore level was long or if the pore mouths were constricted, for example, due to a lower ordering of the tetrahedral framework at the secondary surface, as previously postulated by Serrano and coworkers [25] on the basis of a solid-state nuclear magnetic resonance study. Relating mesopore quality to catalyst lifetime The critical impact of mesopore quality on the lifetime of the ZSM-5 zeolites was revealed in the conversions of methanol (MTH) and of propanal to hydrocarbons, reactions that proceed via mechanistically distinct pathways over protonated ZSM-5 zeolites [12] , [24] . As expected, the conventional zeolites suffered from a sharp deactivation in the conversion of methanol after about 24 h on stream ( Fig. 4a ), which occurred earlier in Z40-C than Z50-C in agreement with the higher concentration of Brønsted acid sites [12] , [46] . Comparatively, the cycle extensions (between two and four times) evidenced over the hierarchical H1 samples, describing the increased length of time for which the conversion exceeded 95%, were typical of those previously reported over ZSM-5 zeolites modified by base leaching [9] , [13] . In stark contrast, despite exhibiting equivalent bulk acidic and porous properties to the H1 zeolites, only minor improvements in the cycle time resulted over the H2 zeolites. 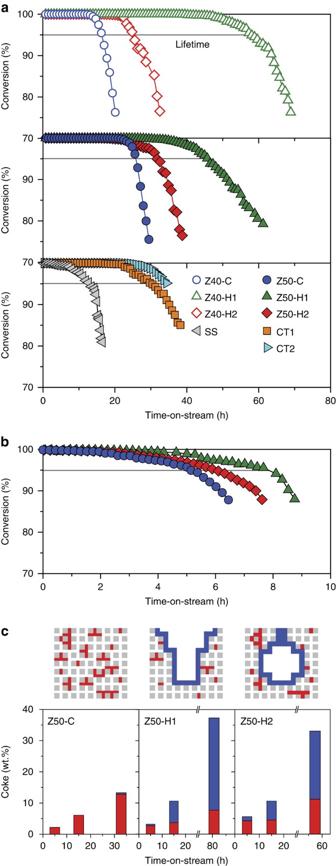Figure 4: Catalytic evaluation. (a,b) The decisive impact of the mesopore quality on the performance of hierarchical zeolite catalysts is unambiguously revealed on evaluation in the conversion of methanol (a) or of propanal (b) to hydrocarbons. The open and well-connected mesopores of the hierarchical H1 zeolites clearly enhance the lifetime (the time for which the conversion exceeds the 95% threshold as indicated, grey line) in comparison with the constricted mesopores in the H2 zeolite, which shows little improvement from that of the conventional ZSM-5. The lower mesopore surface area in the carbon-templated CT zeolites results in limited lifetime benefits, while the intercrystalline mesopores in the SS zeolite prepared by seed silanization also appear to play a spectator role towards the resistance to deactivation in the MTH reaction. (c) The relative lifetime of Z50-H2 with respect to Z50-H1 can be explained by the increased fraction of coke deposited within the micropores (internal, red bars) than in the mesopores (external, blue bars) in the former sample. Conditions of the methanol conversion:T=723 K,P=1 bar,WHSV=9.5 gmethanolgzeolite−1h−1. Conditions of the propanal conversion:T=673 K,P=1 bar,WHSV=8.1 gpropanalgzeolite−1h−1. Figure 4: Catalytic evaluation. ( a , b ) The decisive impact of the mesopore quality on the performance of hierarchical zeolite catalysts is unambiguously revealed on evaluation in the conversion of methanol ( a ) or of propanal ( b ) to hydrocarbons. The open and well-connected mesopores of the hierarchical H1 zeolites clearly enhance the lifetime (the time for which the conversion exceeds the 95% threshold as indicated, grey line) in comparison with the constricted mesopores in the H2 zeolite, which shows little improvement from that of the conventional ZSM-5. The lower mesopore surface area in the carbon-templated CT zeolites results in limited lifetime benefits, while the intercrystalline mesopores in the SS zeolite prepared by seed silanization also appear to play a spectator role towards the resistance to deactivation in the MTH reaction. ( c ) The relative lifetime of Z50-H2 with respect to Z50-H1 can be explained by the increased fraction of coke deposited within the micropores (internal, red bars) than in the mesopores (external, blue bars) in the former sample. Conditions of the methanol conversion: T =723 K, P =1 bar, WHSV =9.5 g methanol g zeolite −1 h −1 . Conditions of the propanal conversion: T =673 K, P =1 bar, WHSV =8.1 g propanal g zeolite −1 h −1 . Full size image Until now, the resistance of hierarchical zeolites to deactivation by coking has been most convincingly correlated with the increased external surface area [11] . However, the prominent differences in the lifetime of the H1 and H2 zeolites demonstrate that the effectiveness of auxiliary mesopores does not exclusively depend on this parameter ( Fig. 5a ). It has also been suggested that the performance is strongly linked with the number of internal defects in the zeolite crystals [47] , [48] . To evaluate this possibility, we estimated the defect concentrations in the samples from the ratio of the infrared absorbance corresponding to isolated internal silanol groups (associated with framework defects) and to terminal silanol groups at the external surface ( I 3726 / I 3745 ), but no satisfactory correlation was observed with the catalyst lifetime in the MTH reaction ( Supplementary Fig. 6 ). While internal defects are likely to promote coke formation, their removal by base leaching does not appear to be beneficial in the case of the H2 zeolites, suggesting that the provision of accessible mesopore surface has a dominant impact. At the same time, an improved description of the catalyst lifetime could be attained with the fraction of o -Ps annihilating in vacuum ( Fig. 5b ), indicating that the global connectivity of the intracrystalline pore network can significantly impact the potential enhancement achievable through hierarchical structuring. A general correlation was also observed with the accessible mesopore volume ( Fig. 5c ). However, neither of these parameters provides a universal descriptor of the catalyst lifetime for all the samples. In particular, the high amount of o -Ps decaying in vacuum evidenced in a fresh Z40-H2 with the partially constricted mesopores does not account for the rapid loss of their function during the MTH reaction. 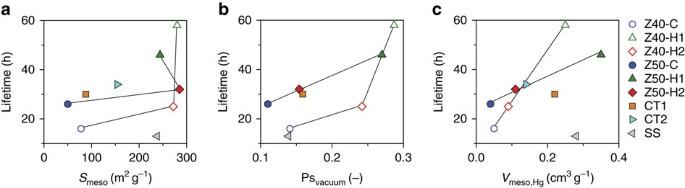Figure 5: Descriptors of the methanol to hydrocarbons performance of hierarchical zeolites. (a–c) Comparison of different structure-performance relationships clearly reveals that the catalyst lifetime is not solely governed by the mesopore surface area of the zeolites (a), but actually strongly depends on the connectivity of the mesopore network as described by the amount ofo-Ps escaping into vacuum derived by PALS (b) and by the mesopore volume accessible to mercury (c). However, while both these parameters provide an indicator of the openness of the mesopores, they are not linearly correlated: the relative fraction ofo-Ps decaying in vacuum is more significantly increased than the accessible mesopore volume in the presence of small mesopores (that is <4 nm in Z40-H2); while the reverse is true in the presence of intercrystalline mesopores such as those displayed in SS zeolite, leading to deviations with respect to the measured catalyst lifetime. The lines are shown for guidance only. Figure 5: Descriptors of the methanol to hydrocarbons performance of hierarchical zeolites. ( a – c ) Comparison of different structure-performance relationships clearly reveals that the catalyst lifetime is not solely governed by the mesopore surface area of the zeolites ( a ), but actually strongly depends on the connectivity of the mesopore network as described by the amount of o -Ps escaping into vacuum derived by PALS ( b ) and by the mesopore volume accessible to mercury ( c ). However, while both these parameters provide an indicator of the openness of the mesopores, they are not linearly correlated: the relative fraction of o -Ps decaying in vacuum is more significantly increased than the accessible mesopore volume in the presence of small mesopores (that is <4 nm in Z40-H2); while the reverse is true in the presence of intercrystalline mesopores such as those displayed in SS zeolite, leading to deviations with respect to the measured catalyst lifetime. The lines are shown for guidance only. Full size image In the conversion of propanal, similar deactivation behaviour was observed over the demetallated zeolites to that evidenced in the MTH reaction ( Fig. 4b ). However, in this case the loss of activity with time on stream occurred more rapidly in agreement with the fast deactivation reported previously by Resasco and coworkers [23] , [24] . The linear correlation established between the catalyst lifetime and Ps vacuum or V meso, Hg emphasized the wider significance of the findings for other organic transformations. Analysis of the intrinsic activity, selectivity and the coking rate of the catalysts further demonstrated the key role of mesopore quality in extending the lifetime of hierarchical zeolites. When the methanol loading was increased to reach conversions <100%, almost identical initial activities were evidenced over the C, H1 and H2 zeolites ( Supplementary Fig. 7 ). However, the initial deactivation rate, which is linked to the rate of coking in the reaction studied, was higher over the alkaline-treated catalysts in comparison with the conventional zeolite, which correlates well with the higher amount of coke deposited over these samples after 5 h of reaction ( Fig. 4c ). Accordingly, the purely microporous zeolites are less prone to deactivation than the hierarchical counterparts, emphasizing the dominance of the mesoporosity for the lifetime prolongation. It is noteworthy that the differing mesopore topology within the zeolites did not significantly impact the product distribution ( Supplementary Table 2 ). In comparison with their conventional counterparts, a marginally higher selectivity to C 5 -C 7 alkanes, compensated by slightly decreased selectivity to C 6 -C 8 aromatics, C 1 -C 4 alkanes and/or C 2 -C 4 olefins was observed over the demetallated zeolites under the conditions studied. Analysis of the relative proportions of coke deposited within the micropores (internal) or the mesopores (external) of the catalysts, based on the variation in porous properties with time-on-stream ( Supplementary Fig. 8 ), provided further insight into the influence of the mesopore organization on the deactivation behaviour. It should be recalled that in reality an axial distribution of coke exists within the catalyst bed [49] , [50] , and consequently the porosity alterations derived by gas sorption correspond to the average impact. Nevertheless, the considerably larger amount of internal coke evidenced over the conventional zeolite (close to 100% after 15 h on stream) in comparison with the demetallated H1 zeolites (<20% in the spent catalyst) clearly demonstrates the beneficial impact of intracrystalline mesopores in preserving the accessibility of the micropores, which is in line with previous findings [10] , [11] . The lower amount of internal coke in the H1 zeolites than in the H2 zeolite (34%) at the end of the cycle further illustrates the essential requirement for open mesopores to minimize the rate of micropore blockage and subsequent deactivation. Complementary characterization by PALS ( Table 2 ) showed that the fraction of o -Ps decaying in vacuum progressively decreased with time-on-stream, which interestingly reached similar values for the catalysts recovered at the end of the MTH cycle. At the same time, the contribution of o -Ps annihilating in the mesopores increased in the H1 zeolite consistent with the progressive blockage of mesopores by the coke deposited. For the H2 zeolites, this value was originally higher due to the presence of constricted mesopores and remained fairly constant during the reaction. Similarly only a minor change in the mesopore volume determined by mercury was observed ( Supplementary Fig. 8 ). Finally, it is worth mentioning that the reusability of the H1 zeolites was confirmed by the equivalent lifetime observed during a second cycle following oxidative regeneration in air (823 K, 5 h). The preserved performance can be expected given the high (hydro)thermal stability of this material, which we have confirmed by thermal (1,223 K, N 2 flow, 5 h) and steam (1,023 K, 30 cm 3 min −1 N 2 flow, H 2 O partial pressure of 300 mbar, 5 h) treatments. The fact that no significant alteration of the porosity or crystallinity was evidenced highlights the robustness of highly mesoporous ZSM-5 zeolites prepared by desilication. Comparative evaluation of the hierarchical CT1 and SS zeolites in the MTH in the MTH reaction revealed lifetimes of 30 and 13 h, respectively, bringing little or no benefit with respect to the purely microporous ZSM-5 ( Fig. 4a ). These results could be ascribed to the low acid site concentrations as well as the poor mesopore network quality, evidenced by pyridine adsorption and PALS, respectively. The former is also responsible for the almost 30% lower initial activity ( Supplementary Fig. 7 ) and increased selectivity to C 2 -C 4 olefins ( Supplementary Table 2 ) observed over these catalysts. It is of note that the fraction of o -Ps annihilating in vacuum still provides a reasonable descriptor of the MTH lifetime ( Fig. 5b ). Furthermore, in the case of the zeolite prepared by seed silanization, the similar pore network connectivity determined by PALS coincides with the preferential deposition of coke in the micropores (93% after 20 h on stream) analogous to that of the conventional zeolite. Interestingly, despite exhibiting distinct mesopore surface area and number of Brønsted acid sites, the carbon-templated CT1 and CT2 zeolites displayed almost equivalent catalyst lifetime, indicating that another property, such as the mesopore quality, is controlling the performance. We have demonstrated the major impact of mesopore architecture on the function of hierarchical zeolite catalysts. A strategic approach exploiting additives during alkaline-mediated demetallation was adopted to spatially manipulate the creation of mesopores within zeolite crystals. The positional and topological assessment of the mesopores, fundamental to establish the concept of mesopore quality, was enabled by the identification of suitable characterization tools. In particular, complementary to high-resolution TEM studies, identical-location scanning transmission and secondary electron microscopy uniquely resolved the highly preserved crystal surface constricting the access to the internal mesopores formed on application of the tetrapropylammonium bromide additive. Positron annihilation lifetime spectroscopy, applied for a first time to characterize the complex pore network of hierarchical zeolites, provided a means of gauging the failure of the constricted mesopores to enhance the connectivity of the intrinsic micropores with the crystal surface. These findings enabled us to quantify the implications of ‘good’ or ‘bad’ hierarchical structuring for the longevity of zeolite catalysts in the conversion of methanol and of propanal to hydrocarbons. Extended lifetimes resulted from the presence of open and interconnected mesopore structures rather than smaller constricted mesopores, which was closely correlated with the fraction of positronium emitted into vacuum derived by PALS and with the relative mesopore volume penetrable by mercury. Juxtaposition of the mesopore quality of hierarchical zeolites prepared by demetallation with those synthesized by carbon templating or seed silanization was hampered by the difficulty of attaining samples with matching characteristics. The variable catalytic benefits observed for the zeolites attained by direct synthesis, highlighted the complex interplay between the mesopore and acid site quality. These findings evidence the importance of assessing the mesopore network attributes beyond standard porosity characterization to design superior zeolite catalysts. Hierarchical zeolite preparation The conventional zeolites (CBV 8014 from Zeolyst International, nominal Si/Al=40, coded Z40-C and PZ-2/100 from Zeochem, nominal Si/Al=50, coded Z50-C) were calcined at 823 K (5 K min −1 ) for 5 h to obtain the protonic form. Alkaline-treated ZSM-5 with distinct intracrystalline mesoporosity was prepared by treating the conventional zeolites in aqueous sodium hydroxide (0.2 M, 30 cm 3 per gram of zeolite) at 338 K, in the absence (coded Z40-H1 and Z50-H1) or presence (coded Z40-H2 and Z50-H2) of tetrapropylammonium bromide (0.2 M). After 30 min, the slurries were quenched and the solids collected by filtration, washed and dried for 10 h at 338 K. Carbon-templated ZSM-5 (coded CT1) was synthesized following an established protocol [19] , in which carbon black particles (5 g, BP-2000, Cabot Corporation) were impregnated with a mixture of tetrapropylammonium hydroxide (8.6 g, 40 wt%), sodium aluminate (0.1 g), ethanol (7.6 g) and water (1.3 g). After evaporation of ethanol at room temperature for 12 h, tetraethoxysilane (9.7 g) was added. The impregnated carbon was hydrolysed overnight, then placed into a Teflon-lined stainless steel autoclave containing 50 cm 3 of water and kept at 453 K for 3 days. The resulting solids were filtered, washed and dried at 383 K for 10 h. The carbon black was removed by controlled combustion in an air flow at 823 K (2 K min −1 ) for 20 h. In addition, a reference carbon-templated sample (coded CT2) was kindly supplied by Haldor Topsøe. Synthesis of hierarchical ZSM-5 via seed silanization (coded SS) was conducted according to a protocol published elsewhere [21] . A precursor solution containing tetraethoxysilane (23.8 g), tetrapropylammonium hydroxide (5.7 g, 40 wt%), aluminium isopropoxide (0.5 g) and water (68.5 g) was aged under reflux at 333 K for 20 h. The resulting protozeolitic units were functionalized with phenylaminopropyltrimethoxysilane (12 mol% with respect to the silica content) at 333 K for 24 h in the presence of 2-propanol, using an organosilane/alcohol weight ratio of 0.076. The majority of 2-propanol was subsequently removed by rotary evaporation, and the final mixture was crystallized in an autoclave under static conditions at 443 K for 7 days. The resulting solid was separated by filtration, washed, dried at 338 K for 10 h, and calcined at 823 K (2 K min −1 ) for 5 h. All the as-synthesized hierarchical zeolites were converted to the ammonium form by three consecutive treatments in aqueous ammonium nitrate (0.1 M, 338 K, 6 h, 100 cm 3 per gram of zeolite) and finally calcined at 823 K (5 K min −1 ) for 5 h to yield the protonic form. Characterization methods X-ray diffraction (XRD) was undertaken using a PANalytical X’Pert PRO-MPD diffractometer operated in Bragg-Brentano geometry using Ni-filtered Cu K α radiation ( λ =0.1541, nm). Data were recorded in the range of 5–50° 2 θ with an angular step size of 0.05° and a counting time of 8 s per step. Inductively coupled plasma-optical emission spectroscopy was conducted using a Horiba Ultra 2 instrument. Nitrogen sorption at 77 K was performed using a Quantachrome Quadrasorb SI after sample evacuation at 573 K for 8 h. Mercury intrusion porosimetry was undertaken with a Micromeritics Autopore IV 9510 following in situ sample evacuation. Transmission electron micrographs were acquired using a Philips Tecnai F30 microscope operating at 300 kV. Correlative STEM was performed on an aberration-corrected Hitachi HD2700C operated at 200 kV and equipped with a secondary electron detector. Infrared spectroscopy of adsorbed pyridine was undertaken using a Bruker IFS 66 spectrometer. Self-supporting zeolite wafers (1 mm 2 ) were degassed at 10 −3 mbar and 693 K for 4 h before analysis. Following adsorption at room temperature, weakly bound pyridine molecules were evacuated at 473 K for 30 min. The concentrations of Brønsted and Lewis acid sites were determined using extinction coefficients of ε(Brønsted)=1.67 cm μmol −1 and ε(Lewis)=2.94 cm μmol −1 . The temperature-programmed surface reaction (TPSR) of n -propylamine was undertaken using a Micromeritics AutoChem 2920 and MKS Cirrus 2 residual gas analyser. Following in situ pretreatment in flowing He (50 cm 3 min −1 ) at 773 K for 2 h, the samples were saturated with n -propylamine at 473 K. Physisorbed amine was removed by purging with He. Decomposition of n -propylamine was monitored in the range 473–773 K using a heating rate of 10 K min −1 . A matrix deconvolution procedure was applied to separate the mass spectrum signals for n -propylamine, propene and ammonia. Positron annihilation lifetime spectroscopy (PALS) was undertaken using the ETHZ slow positron beam (pictured in Supplementary Fig. 9 ) [51] . The powdered zeolites were degassed in situ under vacuum at 295 K for 2 h. Monoenergetic positrons were accelerated into the sample under low-energy conditions (10 keV), resulting in a mean implantation depth of 1,000 nm [52] . The PALS spectra were best fitted by six exponential lifetime components. Their relative fractions were extracted using a fitting method based on Markov chain Monte-Carlo Bayesian inference calculations in the PAScual data suite [53] after subtraction of the background due to accidentals, that is, uncorrelated start-stop signals. The fitting procedure is fully detailed in Supplementary Methods and Supplementary Figs 10 and 11 . The calculated diameters of mesopores were corrected for the effect of the ortho-positronium escaping into vacuum, which reduces the effective lifetime in the mesopores [54] . In contrast, due to the complexity involved, this model did not account for the possible trapping of ortho-positronium in occluded pores. Coke contents in the used catalysts were quantified by thermogravimetric analysis in air using a Mettler Toledo TGA/DSC 1 system with a heating ramp of 10 K min −1 . The proportion of internal coke was estimated from the decrease in micropore volume compared with the starting zeolite, assuming a coke density of 1.22 g cm −3 . The amount of external coke was calculated from the difference between the total and internal coke content [55] . Catalytic testing The methanol-to-hydrocarbon (MTH) reaction was studied at 723 K at ambient pressure using a continuous flow fixed-bed reactor (13.5 mm i.d.) in a Microactivity Reference unit (PID Eng & Tech). The zeolites (0.5 g, particle size=0.2–0.4 mm, diluted with 1.5 g silicon carbide) were pretreated under a nitrogen flow at 723 K for 30 min. Liquid methanol (99.9%) was fed into the preheating zone of the reactor using an HPLC pump, where it was subsequently vapourized in a nitrogen flow (48.9 cm 3 min −1 ) to achieve the desired weight hourly space velocity ( WHSV =9.5 g methanol g zeolite −1 h −1 ). The gaseous products were analysed using an on-line Agilent 7890A gas chromatography equipped with a HP-PLOT Q column and a flame ionization detector (FID). Both methanol and dimethylether were considered as reactant species in calculating the conversion. The intrinsic activity of the zeolites was evaluated by increasing the WHSV to 118.8 g methanol g zeolite −1 h −1 . The conversion of propanal was studied at 673 K at ambient pressure in a continuous-flow fixed-bed reactor (12 mm i.d.). The catalyst (0.3 g, particle size=0.2–0.4 mm) was pre-treated as described above. Propanal was fed into the reactor using a syringe pump via a vapourization line and diluted with He (50 cm 3 min −1 ) resulting in WHSV =8.1 g propanal g zeolite −1 h −1 . The products were analysed with an on-line Agilent 6890 GC system equipped with a HP-5 column and FID. In both reactions, the catalyst lifetime was defined as the duration of a single catalytic cycle, defined as the time-on-stream for which the conversion exceeds 95%. How to cite this article: Milina, M. et al. Mesopore quality determines the lifetime of hierarchically structured zeolite catalysts. Nat. Commun. 5:3922 doi: 10.1038/ncomms4922 (2014).